The European functional tree of bird life in the face of global change Despite the recognized joint impact of climate and land cover change on facets of biodiversity and their associated functions, risk assessments have primarily evaluated impacts on species ranges and richness. Here we quantify the sensitivity of the functional structure of European avian assemblages to changes in both regional climate and land cover. We combine species range forecasts with functional-trait information. We show that species sensitivity to environmental change is randomly distributed across the functional tree of the European avifauna and that functionally unique species are not disproportionately threatened by 2080. However, projected species range changes will modify the mean species richness and functional diversity of bird diets and feeding behaviours. This will unequally affect the spatial structure of functional diversity, leading to homogenization across Europe. Therefore, global changes may alter the functional structure of species assemblages in the future in ways that need to be accounted for in conservation planning. Both climate and land cover change are the major causes of the current unprecedented rates of global biodiversity loss that may, ultimately, deteriorate the structure of biota [1] , ecosystem stability [2] and ecosystem service provisioning [3] . Indeed, the current and future response of species to climate and land use changes can substantially have an impact on species assemblages and, therefore, alter phylogenetic and functional structures [4] . When evaluating how changes in land cover and regional climate might impinge on biodiversity, focus on facets of biological diversity that go beyond the commonly studied species richness or turnover is crucial [4] . Phylogenetic diversity (PD) in species assemblages is, for instance, important for explaining the role of species interactions and biogeographic histories in structuring communities [5] . Further, functional diversity (FD), reflecting the diversity of morphological, physiological and ecological traits within biological assemblages [6] better depicts ecosystem functions and associated services than simple patterns of species richness and turnover [7] . Beyond aesthetic, patrimonial and philosophical arguments, the maintenance of FD is a powerful argument to halt the so-called sixth extinction [3] . Loss of functions provided by particular species, if these are forced to relocate or to become locally extinct due to changes in land cover or climate, likely jeopardizes important regional ecosystem processes [8] . This underscores the importance of quantifying how functional uniqueness and diversity of species assemblages relates to the projected sensitivity of species to environmental changes. Not all species are equally influenced by changes in climate or land cover. Generalist species are often perceived as being less sensitive to such changes than specialists that have traits adapted to a narrower range of conditions [9] . Indeed, a recent modelling study on Alpine plants indicates lower extinction risk for generalists compared with rare and threatened plant species [10] . Increase in forests, agriculture and urban areas at the expense of semi-natural grasslands, together with change in precipitation regimes and temperature increase, may influence the structure of avian assemblages [11] and their associated FD. Bird assemblages are interesting to study as they heavily depend on both vegetation structure and climate, and have been shown to have important ecological role on ecosystem functioning and associated services [12] . Through their mutualisms with plants, birds act as genetic linkers by pollinating flowers and transporting seeds, thereby helping to maintain plant diversity by supporting gene flow [12] , [13] . Scavengers on carcasses help to limit disease spread while predators on vertebrates and insects play important roles in the regulation of prey density [12] , [13] , [14] . As another example, cavity-drillers and nest-burrowers are recognized as ecosystem engineers that provide shelter to additional species [13] , [15] , [16] . Beside these direct functions, birds also provide important cultural services for nature enthusiasts and contribute to global nutrient dynamics [13] . Climate- or land cover-induced modifications in bird assemblages could have cascading negative effects in trophic chains, and strongly reduce the provision of some functions. For instance, a decline in top predators could benefit prey species, with radiating effects on all lower trophic levels [17] , [18] . Therefore, biological simplification of agricultural lands or forests through land use intensification may decrease the provisioning of pest control and other ecosystem services by birds if their taxonomic and FD decline [15] , [19] . Moreover, if global changes lead to more homogenous landscapes, then this naturally translates into more similar animal assemblages [20] . Functionally diverse assemblages likely show greater complementarity in resource use and thus provide enhanced ecosystem functioning [21] . Alternatively, assemblages with numerous similar species have a greater chance to provide more functional insurance against environmental changes (for example, pesticides or diseases) than functionally diverse assemblages because redundancy buffers against loss of functions otherwise provided by single species [22] . Although these specific threats are difficult to account for or predict, it is nevertheless crucial to project the potential detrimental or beneficial effects on FD by projected climate and land cover change at large spatial scales [23] . Here we report impact analyses of changes in land cover and regional climate on the distribution of 402 European breeding bird species and the resulting effects on the FD of bird assemblages. FD is represented here by behavioural traits during feeding to reflect how species acquire resources from their environment (feeding behaviour, feeding location and activity), and by body mass and diet traits to reflect the resource use requirements of species. We consider these as effect traits that determine the impact of a given organism on community structure and ecosystem functioning [24] , [25] , although the distinction between effect and response traits (traits that stand for the response of organisms to environmental change) is not always straightforward for animals [14] . In order to project current and future suitable habitats for each species, we use consensus projections extracted from multiple species distribution models, several up-to-date high-resolution regional climate models and land cover change scenarios, where the latter two originate from recently finished EU projects. First, we ask whether species sensitivity to climate and land cover change is randomly distributed across a functional tree of the European avifauna, depicted as a dendrogram based on interspecific functional distances. Second, we test whether functionally unique species (species bearing singular combination of traits) are projected to experience more-severe changes in suitable climates and habitats than species bearing more common trait syndromes. Third, we ask whether changes in species habitat suitability influence the richness (that is, the number of species bearing each function) and FD of different guilds. To do so, we investigate species richness and FD in diet, feeding behaviour and location, and activity and body mass over Europe. By investigating whether the FD in feeding behaviour and location within each diet type (and similarly for the other trait types) responds to global change, we identify the functions that will likely increase or decrease in frequency and diversity. Finally, we test for spatial structure in expected change of FD. To this end, we map current and future FD of bird assemblages, and we investigate spatial changes in regional FD across Europe. Under the assumptions that bird species will track their suitable climate and land cover, we showed that species bearing unique trait combinations were not more sensitive than other species, and that the trait diversity of some guilds was projected to change drastically (that is, insectivores) while other guilds should not be strongly affected. Overall, the spatial distribution of trait diversity should change across Europe, leading to functional homogenization of its avifauna. Species sensitivity to climate and land cover changes Species sensitivity to both climate and land use change is estimated as the change in the amount of suitable habitat assuming that all species fully disperse to newly suitable habitats and track their shifting niche without any response lag. Most species are predicted to shift their range North- and up-ward [11] , with a moderate increase in the amount of suitable habitat for most species under the A1B scenario ( Fig. 1a ; Supplementary Fig. 1 for the other regional climate and land cover scenarios). This implies that, although several species are predicted to lose a substantial part of their current suitable habitat ( Fig. 1b ; Supplementary Fig. 1B ), the majority is predicted to find larger extents of suitable habitat elsewhere in Europe under future conditions ( Fig. 1a ; Supplementary Fig. 1A ). 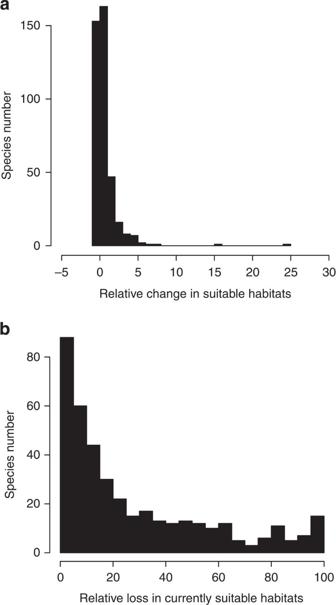Figure 1: Distribution of changes in suitable habitats and loss in currently suitable habitats. Histograms representing the projected relative change in suitable habitats (a) and loss in currently suitable habitats (b) (in percentage) under the A1b emission scenarios by 2080, using the RCA30 regional climate model driven by the ECHAM5 global circulation model and ensembles of five species distribution models. Theyaxis represents the number of species for each class of projected change in suitable habitats. Ina, most of species are projected to experience between −2% and +5% of change in suitable habitats (with negative values standing for a loss in suitable habitat while positive values are a gain). Figure 1: Distribution of changes in suitable habitats and loss in currently suitable habitats. Histograms representing the projected relative change in suitable habitats ( a ) and loss in currently suitable habitats ( b ) (in percentage) under the A1b emission scenarios by 2080, using the RCA30 regional climate model driven by the ECHAM5 global circulation model and ensembles of five species distribution models. The y axis represents the number of species for each class of projected change in suitable habitats. In a , most of species are projected to experience between −2% and +5% of change in suitable habitats (with negative values standing for a loss in suitable habitat while positive values are a gain). Full size image Species sensitivity distribution along the functional tree Among European bird species, we find only a weak, nonsignificant relationship between relative changes in the size of suitable habitat area following climate and land cover change and the position of species on the functional tree ( Fig. 2 ; Supplementary Fig. 2 and Supplementary Table 1 ). This demonstrates that no group of functionally similar species is predicted to be particularly sensitive or insensitive to global change. This is surprising since large body mass and other life history traits usually predispose species to increased extinction risks [26] . 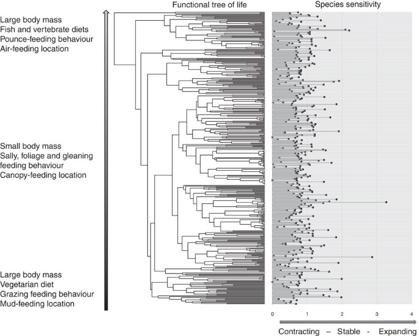Figure 2: Link between the European functional tree of bird life and species sensitivity to climate change. Species sensitivity measured as change in suitable habitat and mapped on the functional tree of the avifauna for one emission scenario (A1B) by 2080, using the RCA30 regional climate model driven by the ECHAM5 global circulation model and ensembles of five species distribution models. Species sensitivity was log-transformed (log(CHS-1-min(CHS)) for this analysis. Importantly, functionally unique species are unlikely more sensitive to environmental change than are functionally less unique species ( Supplementary Table 2 ). The functional uniqueness of species is therefore not clustered on the phylogenetic tree of the European avifauna ( Fig. 3 ). Figure 2: Link between the European functional tree of bird life and species sensitivity to climate change. Species sensitivity measured as change in suitable habitat and mapped on the functional tree of the avifauna for one emission scenario (A1B) by 2080, using the RCA30 regional climate model driven by the ECHAM5 global circulation model and ensembles of five species distribution models. Species sensitivity was log-transformed (log(CHS-1-min(CHS)) for this analysis. 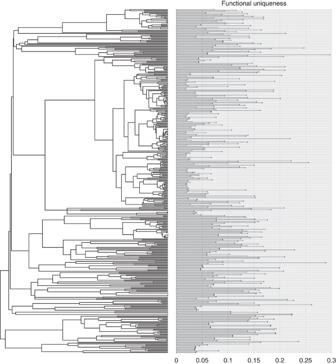Figure 3: Functional uniqueness of the European avifauna mapped on the phylogenetic tree63. There was no significant phylogenetic signal of functional uniqueness (Pagel’s lambda likelihood ratio testP>0.05 (ref.61)). Functionally unique species were not more closely related to each other than if sampled randomly along the phylogeny. Full size image Figure 3: Functional uniqueness of the European avifauna mapped on the phylogenetic tree [63] . There was no significant phylogenetic signal of functional uniqueness (Pagel’s lambda likelihood ratio test P >0.05 (ref. 61 )). Functionally unique species were not more closely related to each other than if sampled randomly along the phylogeny. Full size image Change in richness and diversity across functional groups Interestingly, the projected species richness and FD within each of the five groups of analysed traits (diet, feeding behaviour, feeding location, feeding activity and body mass) show diverging patterns in response to environmental changes ( Fig. 4 for diet, Fig. 5 for feeding behaviour and Supplementary Figs 3–5 for the other traits). Whereas the mean and variance in body mass per pixel did not significantly change ( Supplementary Fig. 5 ), there was a noticeable increase in the mean species richness of invertebrate diet and picking and pecking feeding behaviour with environmental change. Interestingly, this increase in species richness for these two specific diet and feeding behaviour groups is not followed by an increase in FD (as measured by mean pair-wise functional distance (MFD)), whether or not we consider all traits or single traits. In other words, the increase in species richness for the invertebrate diet will not result in a higher diversity in feeding behaviour or feeding locations. This is because all of these behaviours are already represented within each pixel. In summary, our results reveal an increase in redundancy for invertebrate diet and picking and pecking feeding behaviour. On the contrary, other diet groups are projected to experience an increase in species richness per pixel, while their FD is projected to decline at the same time ( Fig. 4 ) such as, for instance, bird assemblages with a vertebrate diet. The diversity of feeding behaviours within the vertebrate diet group is projected to slightly decrease, resulting in a decrease in complementarity. In contrast, the fish diet group is projected to experience decreased FD in feeding behaviours and locations, without an associated change in species richness. 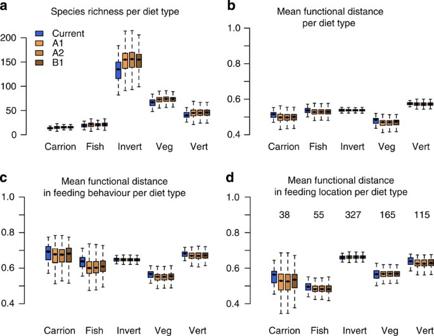Figure 4: Species richness and functional diversity per diet type across Europe under current and three future climate and land cover scenarios. Each bar of the boxplot (sample size =402 species) represents the median, first and third quartiles (defining the filled box) and minimum and maximum values (error bars excluding outliers) of the distributions of: species richness (a), MFD considering all remaining traits except diet (b), MFD considering feeding behaviour only (c) and MFD considering feeding location only (d) mapped over Europe. Theyaxis represents the number of species (a) and the MFD values per functional group (b–d). Colour code is indicated ina. Species number per feeding behaviour is indicated ind. Only projections for climatic scenarios by 2080 and modelled under the RCA30 regional climate model are represented. The influence of regional climate models is represented inSupplementary Fig. 8. Figure 4: Species richness and functional diversity per diet type across Europe under current and three future climate and land cover scenarios. Each bar of the boxplot (sample size =402 species) represents the median, first and third quartiles (defining the filled box) and minimum and maximum values (error bars excluding outliers) of the distributions of: species richness ( a ), MFD considering all remaining traits except diet ( b ), MFD considering feeding behaviour only ( c ) and MFD considering feeding location only ( d ) mapped over Europe. The y axis represents the number of species ( a ) and the MFD values per functional group ( b – d ). Colour code is indicated in a . Species number per feeding behaviour is indicated in d . Only projections for climatic scenarios by 2080 and modelled under the RCA30 regional climate model are represented. The influence of regional climate models is represented in Supplementary Fig. 8 . 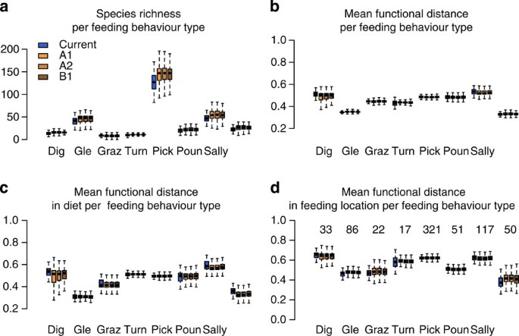Figure 5: Species richness and functional diversity per feeding behaviour type across Europe under current and three future climate and land cover scenarios. Each bar of the boxplot (sample size =402 species) represents the median, first and third quartiles (defining the filled box) and minimum and maximum values (error bars excluding outliers) of the distributions of: species richness (a), MFD considering all remaining traits except feeding behaviour (b), MFD considering diet only (c) and MFD considering feeding location only (d) mapped over Europe.yaxis represents the number of species (a) and the MFD values per functional group (b–d). Colour code is indicated ina. Species number per feeding behaviour is indicated ind. Only projections for climatic scenarios by 2080 and modelled under the RCA30 regional climate model are represented. Dig=digging, Gle=foliage-gleaning, Graz=grazing, Turn=overturning, Pick=picking/pecking/stabbing, Poun=pouncing, Sally=sally. The influence of regional climate models is represented inSupplementary Fig. 8. Full size image Figure 5: Species richness and functional diversity per feeding behaviour type across Europe under current and three future climate and land cover scenarios. Each bar of the boxplot (sample size =402 species) represents the median, first and third quartiles (defining the filled box) and minimum and maximum values (error bars excluding outliers) of the distributions of: species richness ( a ), MFD considering all remaining traits except feeding behaviour ( b ), MFD considering diet only ( c ) and MFD considering feeding location only ( d ) mapped over Europe. y axis represents the number of species ( a ) and the MFD values per functional group ( b – d ). Colour code is indicated in a . Species number per feeding behaviour is indicated in d . Only projections for climatic scenarios by 2080 and modelled under the RCA30 regional climate model are represented. Dig=digging, Gle=foliage-gleaning, Graz=grazing, Turn=overturning, Pick=picking/pecking/stabbing, Poun=pouncing, Sally=sally. The influence of regional climate models is represented in Supplementary Fig. 8 . Full size image Current and future trait diversity distribution The spatial distribution of the overall FD (calculated as MFD with all traits included) was calculated on a pixel basis among species that were projected to be present at each time period. Our analyses reveal that the projected FD of the avifauna is not homogenously structured across Europe under current conditions, with northern regions and Atlantic coasts having the largest FD and the European Alps and centre of Iberian Peninsula having the lowest. However, despite these projections, European biogeographic regions are not equally affected ( Fig. 6 ). Under current conditions, northern Europe and the northern UK currently exhibit markedly higher bird FD compared with central Europe (for example, southern Germany), the centre of the Iberian Peninsula and the outer Alps ( Fig. 6 ). Under projected global change, however, the marked difference between Northern and central Europe tends to be reduced. In particular, mountainous regions of central and southern Europe are projected to experience marked increase in FD. For southern Scandinavia (that is, nemoral and boreal regions) we predict reduction in FD in many parts. In other words, the expected upward shift of suitable habitats for European birds in central European mountains may lead to a relative increase in FD (assemblages being functionally less redundant). In contrast, for northern latitudes, we predict assemblages to become functionally more redundant. The simulated differences between the various climate and land cover scenarios are relatively small and do not greatly alter spatial patterns ( Fig. 6 ). In general, under the A1b climatic scenario and the associated GRAS land use scenario, the projected changes are the most marked, with stronger relative increase in FD in the Alps and at centre of the Iberian Peninsula, and stronger relative decrease in northern UK and southern Scandinavia than under the A2 and B1 scenarios ( Fig. 6 ). 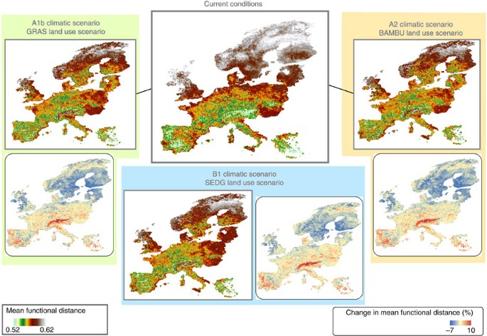Figure 6: Mean pair-wise functional distance and its projected changes across Europe under current and future conditions. Large panels represent the per pixel functional diversity of European avifauna. Small panels show the relative change in functional diversity between future and current conditions. Figure 6: Mean pair-wise functional distance and its projected changes across Europe under current and future conditions. Large panels represent the per pixel functional diversity of European avifauna. Small panels show the relative change in functional diversity between future and current conditions. Full size image The analysis of joint climate and land cover change impact on the FD of an entire species group over large spatial scales are challenging. Our study addresses these challenges and presents an unique large-scale assessment of the potential impacts of combined climate and land cover changes on the FD and richness of European avifaunal assemblages. Our study addresses important drawbacks of most existing global change risk assessments. In methodological terms, our study is one of the first to model the response of species to both regional climate and land use changes. For instance, Thuiller et al. [27] quantified the influence of climate change on the PD of European biota but only focused on climate change as simulated from global (not regional) circulation models and ignored potential additional effects of projected land cover change. As suggested by Barbet-Massin et al. [28] , we estimate the climatic and land cover requirements of species for the whole western Palearctic region including northern Africa. This allows us to account for species that may immigrate to Europe from North Africa, and ensures that the ecological requirements of the modelled species were fully captured. These estimates are consistent with recent analyses on the same group of species [28] and slightly less alarming than previous studies [29] . The divergence from results of Huntley et al. [29] likely originates from inclusion of the southern and eastern range limits of the modelled European bird species in North Africa and the Middle East [28] . In addition, we use the latest release of regional climate models (RCMs) and also include land cover variables that certainly buffer the direct effects of climate change. Finally, we have employed ensemble-forecasting methodologies by combining highly predictive species distribution models ( Supplementary Fig. 6 to generate robust projections and, thus, use four different RCMs and three socioeconomic scenarios in order to incorporate into our projections all recognized sources of uncertainty. In summary, we show that, although the overall functional avian diversity of Europe is expected to only weakly change under projected climate and land cover change, some regions might experience increased functional complementarity (for example, the European Alps), or simply an increase in species richness per guild (for example, Boreal and Nemoral regions). Overall, this reshuffling should lead to a functional homogenization of Europe, with most combinations of traits occurring being available everywhere in the landscape. This result complements the current opinion that the global avifauna is experiencing functional homogenization due to the loss of specialist and proliferation of generalist species [9] . In our case, the causal factors are slightly different as this homogenization is due to a spatial re-structuring of assemblages and, notably, the arrival of species with new combinations of traits in specific regions (that is, artic and alpine) increasing their functional complementarity. Thus, assemblages with projected increases in FD may provide enhanced ecosystem functioning as a result of more efficient resource use, a beneficial effect that is projected to occur primarily in mountain areas. In any case, we show that species richness in a given guild is not predicted to dramatically drop, meaning that no key functional groups (that is, top predator) are predicted to go locally extinct, which could have had important consequences on trophic cascade. Interestingly, our results demonstrating species with unique combinations of traits are not disproportionally sensitive to climate and land cover change mirror a recent analysis carried out for 32 fish species in France [30] . This study evaluates the potential impact of climate change on fish assemblages and reports that those species at high risk of local extinction are not necessarily those bearing the most unique combination of traits. Our results for European birds show the same trend. Having used effect traits instead of response traits might explain this pattern, as there is no a priori reason to believe that particular combinations of effect traits should negatively influence the response of species to environmental change. The projected changes we present may lead to an increase in richness of species with invertebrate diet and pick and peck feeding behaviour, which, in turn, may have an impact on human well-being through the enhancement of natural pest control [31] . Indeed, an increase in richness of species with invertebrate diets would likely benefit pest control and associated ecosystem services, although the regions that need it most (southern European countries with economies that are highly dependent on agricultural yields) are projected to experience reductions in these services [32] . However, our results need to be treated with caution as the overall FD within the invertebrate diet group and, more specifically, the diversity of feeding behaviours and locations are not projected to change. In other words, change in the richness of species with an invertebrate diet will most likely result in an increase in predation but not in the variety of predation behaviours and locations. More importantly, some diet groups (for example, vertebrate diet) are likely to experience an increase in the mean species richness across Europe, together with a decrease in diversity of feeding behaviour and location. Other groups, such as fish-eating diet, may experience a decrease in FD that is decoupled from changes in species richness. The outcome of such projected changes on complementarity requires additional analyses in order to deduce regional consequences on ecosystem services. Indeed, the link between traits, ecosystem functioning and ecosystem services is far from trivial [14] and is influenced by quantity of other factors not explicitly modelled here, such as community assembly rules and land use practices. Additionally, our modelling framework does not explicitly account for interspecific competition, which could impede the increase in species richness in some groups. Projected change in species richness is thus likely to be the maximum change when competition within a guild does not influence the pure effects of climate and land use change. However, this is also important to note that at the resolution of our study (10 arc-minutes, roughly 19 km in Europe), the outcome of competitive interactions might be moderate as the spatial heterogeneity and the area of a pixel might buffer competitive exclusion within a guild. Our study thus provides clear evidence that the repercussions of projected climate and land use change on FD of European avifauna assemblages is moderate, despite the likely negative impacts of these changes on individual species ranges [11] . One major beneficial effect of environmental changes relates to the projected increase in species with invertebrate diets, which could ultimately influence pest control, but which could also negatively influence pollination services. These detrimental effects relate to a decrease in FD in Northern Scandinavia that might ultimately reflect reduced ecosystem functioning in an arctic region. However, relatively small changes in FD may be paralleled by high regional turnover of individual species that results in substantial changes in trophic relationships that accompany altered species assemblages [4] . Statistical analyses All analyses have been carried out in the R environment [33] (specific functions within specific package are indicated in brackets). Species distribution data Presence–absence data for all European species were obtained from the EBCC atlas of European breeding birds [34] that we further completed for northern Africa and eastern Europe using geo-referencing and digitizing breeding bird distribution maps from the handbooks of the birds of the Western Palaearctic [35] at a 0.5° resolution. We did not consider seabirds in our analysis as climate and land cover variables may not be the most relevant drivers of the restricted terrestrial distribution of their breeding sites. Moreover, our spatial analysis has focused on projected changes in Europe. Therefore, we considered only those species that have their current breeding ranges at least partly included in Europe and we removed species with less than 20 occurrences for statistical modelling reasons. From the total list of European breeding and resident bird species, we finally retained 402 species. For all modelled species, we considered their whole Western Palaearctic range (including North Africa and the Middle East) in order to model the full extent of their environmental niche [28] . Environmental data Current climate was represented by five bioclimatic variables from the Worldclim database [36] at 0.5° resolution for calibrating the models and 10′ resolution for projecting them. These variables were as follows: temperature seasonality (intra-annual standard deviation * 100), maximum temperature of the warmest month, minimum temperature of the coldest month, precipitation of the wettest month and precipitation of the driest month ( Supplementary Table 3 ). Future climate by 2080 (2051–2080) was represented by a set of RCM runs originating from the ENSEMBLES EU project, which has physically downscaled global circulation model (GCM) data generated for the 4th assessment report of the IPCC [37] . We used three available SRES scenarios [38] for these models, namely A1b, A2 and B1. RCMs downscale the very coarse resolution climate model output of CGMs (usually 1–2° Lat/Lon per grid cell) to a much finer spatial resolution (usually 10–30′ Lat/Lon) on a physical process basis. To this end, an RCM is fed at the study area boundaries by the global output of GCMs in order to provide boundary conditions and global weather input for the downscaling. We have used three different RCMs, namely HadRM3, RCA3 and RACMO2 (refs 39 , 40 , 41 , 42 ), fed by three different GCMs (HadCM3, ECHAM5 and CCSM3) and resulting in four RCM/GCM combinations ( Supplementary Table 4 ). All RCM scenarios were interpolated to the same 10′ spatial resolution for 30-year monthly mean values of temperature and precipitation. On the basis of these monthly values, our five bioclimatic variables of the Worldclim database were calculated for future time steps. Current land cover for the whole Palearctic was represented by GLOBCOVER 2009 ( https://earth.esa.int/web/guest/pi-community ) at 300 m resolution. We up-scaled the data to the resolution of the species distributions (0.5°) and 10′ resolution for projection under current and future conditions by calculating the area fraction of each land cover type within each pixel. We used the level 1 classification (that is, built-up areas, arable lands, permanent crops, grasslands, forests and others) that is consistent with the EU CORINE classification on which the land cover scenarios were based. Bird species distributions are also influenced by the structure of the vegetation. Despite the fact that it is difficult to accurately represent the structure of the vegetation mosaic at 0.5° and 10′ resolutions, we estimated the Simpson diversity index using the fraction of each land cover class as a weighting scheme. Future land cover data were taken from the EU-funded ALARM and ECOCHANGE projects [43] , [44] , [45] . The ALARM land cover change scenarios provide annual fractions of land use for eight main land use/cover categories per 10′ resolution grid cell (that is, % built-up, % cropland, % permanent crops, % grassland, % forest, % biofuels (liquid, non-woody or woody) and % land in succession) and for the period 2006–2080. We then retained the period 2051–2080 to be consistent with the climatic data. The countries covered are those of the EU25 plus Switzerland and Norway. We removed % of biofuel and % of land in succession that were not available for calibrating the models (period 1961–1990). We retained three storylines that are consistent with the climate change scenarios: (1) GRAS–Growth Applied Strategy, in which deregulation, free trade, growth and globalization will be policy objectives actively pursued by governments. Environmental policies will focus on damage repair and limited prevention based on cost benefit calculations. There is no emphasis on biodiversity. This scenario is considered equivalent to A1b; (2) BAMBU (Business-As-Might-Be-Usual) in which policy decisions already made in the EU are implemented and enforced. At the national level, deregulation and privatization continue except in ‘strategic areas’. Internationally, there is free trade. Environmental policy is perceived as another technological challenge. This scenario is considered equivalent to A2; and (3) SEDG (Sustainable European Development Goal) that enhances the sustainability of societal development by integrated social, environmental and economic policies. The scenario aims for a competitive economy and a healthy environment, gender equity and international cooperation. It represents a normative scenario with stabilization of GHG emissions. This scenario is considered equivalent to B1. Given the land cover scenarios were only available for the EU25 plus Switzerland and Norway, species projections into the future were only carried out over those 27 countries. In summary, models were calibrated and projected in time using five bioclimatic variables, five land cover type variables and one land cover diversity variable under four RCMs and three emission scenarios. Functional-trait information Trait information for the 402 modelled birds was extracted from the Handbook of the Birds of the Western Palaearctic [35] . Missing species and data were gathered from species publications and Internet websites treating avifauna. The traits were as follows: body mass, diet (invertebrates, vertebrates, vegetal, fish and carrion), feeding behaviour (pursuit (air and/or aquatic), sally, foliage-gleaning, pouncing, grazing, picking/pecking/stabbing, digging, overturning and probing), feeding location (water, mud, ground, canopy and air) and activity (nocturnal, crepuscular and diurnal). For diet, feeding behaviour, and feeding location and activity, each subcategory was expressed as a binary variable (0 or 1) to make sure that a species could be assigned to several strategies. In our study, we did not consider traits that can only be measured with reference to the surrounding environment, such as nesting habitats. We did so because of the circularity in the methodology as changes in land cover (defining the surrounding environment) are implicitly accounted for in our modelling framework. We preferred to constrain our analyses to a specific set of traits that was relevant to understand the implications of environmental change on community assembly [12] . Species distribution modelling Species distribution models were calibrated over the whole western Palearctic biogeographic zone at a resolution of 0.5° and then projected into the future over EU25 plus Switzerland and Norway at 10′ resolution. By this, we considered the whole Western Palaearctic range (including North Africa and the Middle East) to calibrate models for the full extent of the niches of species [28] and to allow species that currently occur only around the margins of Europe to potentially migrate into the EU25 as the climate becomes suitable. An ensemble of forecasts of species distribution models [46] , [47] was obtained for each of the 402 species. The ensemble included projections with Generalized Additive Models, Boosting Regression Trees, Classification Tree Analysis, Multiple Adaptive Regression Splines and Random Forest. Models were calibrated for the baseline period using 65% random sample of the initial data and evaluated against the remaining 35% data, using the True Skill Statistic (TSS [48] ) and the Area Under the receiver operating characheristic Curve (AUC). This analysis was repeated five times, thus providing a fivefold internal cross-validation of the models ( biomod package [49] in R [33] ). The quality of the models was very high to excellent with an average AUC and TSS of 0.97 and 0.87, respectively ( Supplementary Fig. 6 ), while for the least well-modelled species, the ensemble model quality reached an AUC of 0.93 and a TSS of 0.7, which are traditionally considered as good predictive performance [48] . For each species, we projected the probability of occurrence within each 10′ resolution pixel under both current and future conditions as a weighted sum of occurrence-probability projections made by the five modelling techniques run over five subsamples. This modest downscaling at a scale of 1:3 from models calibrated at 0.5° to 10′ projections has been shown to be well suitable at such spatial extent and resolution [50] . The weighting scheme for building ensembles was proportional to the TSS statistics for each modelling technique and cross-validation (that is, the techniques that delivered the most accurate models had the highest weights). Probabilities of occurrence were further transformed into binary maps using the value that maximized the TSS score as a threshold. Dispersal ability Not all species are expected to disperse at the same rate and distance. However, the information about natal dispersal was not known for all the 402 species. To estimate what could be the uncertainty associated to the non-inclusion of natal dispersal, we gathered the information on natal dispersal for 74 species from Paradis et al. [51] and Barbet-Massin et al. [11] For these 74 species, we then estimated the projected change in habitat suitability accounting for natal dispersal, and further compared them with the ones estimated, assuming no dispersal constraints (change in habitat suitability (CHS)). The results for these 74 species confirmed that the non-inclusion of natal dispersal into the modelling procedure for the 402 species should not change the outcome of the analyses ( Supplementary Fig. 7 ). For the time considered (100 years), most species should be able to reach their suitable habitats in terms of climate and land cover change. Species sensitivity to climate and land use change Each ensemble of species projections for current and future conditions were converted into a metric of species sensitivity [27] . CHS measures the relative change in suitable climate and land use. It corresponds to the total suitable area projected into the future under the assumption of unlimited dispersal minus the total suitable area projected on the current conditions, with the resulting quantity divided by the total suitable area projected on the current conditions. There was no relationship between CHS and the predictive performance of the models ( Supplementary Table 5 ). The metric was averaged across Species × Model × Scenario × RCM combinations. Functional distance and the functional tree of bird life We first log-transformed and normalized body mass prior to all analyses. We used a mixed-variables coefficient of distance that generalizes Gower’s coefficient of distance to allow for the treatment of various types of variables when calculating distances [52] . Euclidean distance was used for body mass, while the Sorensen distance [53] (S7 coefficient of Gower and Legendre [54] , function dist.ktab in ade4 ) was used for binary data types—for example, for each subgroup of diet and feeding behaviour trait. Then, we used hierarchical clustering to build the most reliable dendrogram of all species in functional-trait space, employing an average agglomeration method (UPGMA, function hclust ) [55] . The functional dendrogram expressed 78% of the original distances between species (Mantel correlation between the original distance matrix and the distance matrix from the dendrogram equaled 0.78, P -value <0.001 with 9,999 randomizations, function mantel in vegan [56] ). Functional uniqueness and link with species’ sensitivity We adapted the Evolutionary Distinctiveness index [57] , which measures the relative contributions of species to PD, for use in a functional context. First, for each branch of the functional dendrogram, we estimated a value equal to its length divided by the number of species subtending the branch. The functional uniqueness of a species is simply the sum of these values for all branches from which the species is descending, to the root of the functional dendrogram (function originality in ade4 (ref. 58 ). We calculated the strength of the signal between the functional tree and the measure of species sensitivity estimated for the range of climate and land use projections. We used the robust measure proposed by Abouheif [59] to test for serial independence to detect a functional signal in species sensitivity (function abouheif.moran in ade4 ). We tested the strength of the phylogenetic signal in functional uniqueness using Pagel’s lambda statistic and its associated likelihood ratio test [60] , [61] . To test the link between functional uniqueness and species sensitivity to climate and land use change, we calculated Pearson’s correlation between the functional uniqueness of species and their expected sensitivity to the range of climate and land use projections. Species richness per group and FD We estimated the species richness for each category of each functional trait per pixel. We estimated the mean assemblage body mass per pixel (instead of species richness), given that body mass is a continuous variable. To calculate FD, we used the MFD between all species present in a pixel. This index is a classic metric in community ecology [5] , represents an unbiased estimate of the variance of the trait considered and is not correlated with species richness (function mpd in picante [62] ). This was calculated for all traits together (for example, Fig. 4 ) and also within functional groups. For the latter, we re-calculated the functional distance matrix without the trait considered (for example, diet) and calculated the MFD for all remaining traits ( Fig. 3b ) and for single trait (for example, feeding MFD per diet type, Fig. 3c ) within pixel. We analysed the variability to RCMs for MFD for diet and showed that the results were little sensitive to this variability ( Supplementary Fig. 8 ). For the spatial distribution of MFD, we simply mapped the MFD on the geographic space. Relative change in MFD between current and future conditions was estimated as equation 1: How to cite this article: Thuiller, W. et al. The European functional tree of bird life in the face of global change. Nat. Commun. 5:3118 doi: 10.1038/ncomms4118 (2014).